Spin–orbit proximity effect in graphene The development of spintronics devices relies on efficient generation of spin-polarized currents and their electric-field-controlled manipulation. While observation of exceptionally long spin relaxation lengths makes graphene an intriguing material for spintronics studies, electric field modulation of spin currents is almost impossible due to negligible intrinsic spin–orbit coupling of graphene. In this work, we create an artificial interface between monolayer graphene and few-layer semiconducting tungsten disulphide. In these devices, we observe that graphene acquires spin–orbit coupling up to 17 meV, three orders of magnitude higher than its intrinsic value, without modifying the structure of the graphene. The proximity spin–orbit coupling leads to the spin Hall effect even at room temperature, and opens the door to spin field effect transistors. We show that intrinsic defects in tungsten disulphide play an important role in this proximity effect and that graphene can act as a probe to detect defects in semiconducting surfaces. Graphene is a promising material for both fundamental spin-based transport phenomena and low power-consuming spin-based device applications [1] , [2] . Among the first predictions for graphene was the topological insulator with spin-polarized edge states [3] . Furthermore, room temperature (RT) ballistic charge transport [4] and gate-tunability make graphene an ideal material for spin field effect transistors (FETs) [5] . However, graphene’s extremely weak intrinsic spin–orbit coupling (SOC) [6] makes the experimental observation of these phenomena very challenging. Previous studies have shown that the weak hydrogenation of graphene can significantly enhance the SOC [7] , [8] . However, chemical functionalization introduces disorder and severely limits charge mobility and hence, the spin relaxation length [8] , [9] . Equally important, the hybridization between hydrogen and carbon induces a Rashba type SOC by introducing sp [3] defects thereby breaking the inversion symmetry of the lattice [10] . The decoration of the graphene surface with heavy-metal adatoms such as gold (Au), indium (In) or thallium (Tl) has also been proposed to increase the SOC [11] , [12] . However, also this approach introduces disorder and hence, equally limits both charge and spin transport properties [13] . These challenges have recently brought to light other two-dimensional crystals such as transition metal dichalcogenides (TMDCs). TMDCs have band gaps in a technologically attractive energy range (~1–2 eV) and orders of magnitude higher SOC than graphene [14] . This, combined with spin split bands makes them an almost ideal material for spintronics. However, the presence of unavoidable defects in TMDCs typically limits their electron mobilities to μ ~100 cm 2 V −1 s −1 (ref. 15 ). Hence, we expect a spin relaxation length even lower than in weakly hydrogenated graphene. In this work, we show that by utilizing the proximity effect between graphene and TMDCs one can keep the extraordinary high mobilities of crystalline graphene and at the same time enhance its SOC to allow electric field controllable spin currents at RT. Since graphene and WS 2 have comparable workfunctions (~4.6 eV and ~4.7 eV, respectively) [16] , [17] , [18] , the charge neutrality point of graphene on WS 2 is expected to be located approximately in the middle of the energy gap of WS 2 . Therefore, naively, one would expect WS 2 to act just as another inert substrate, such as SiO 2 or BN. Remarkably, the presence of intrinsic defects in WS 2 creates electronic states that overlap in energy with the electronic states of graphene. Because of the finite thickness of the WS 2 (~10 nm) substrate, the number of these defects is large. Thus, above a threshold back-gate voltage ( V TH ) they act as a sink for electronic charges, resulting in a gate bias ( V BG )-independent conductivity. For V BG < V TH , our devices have electronic mobilities as high as 50,000 cm 2 V −1 s −1 , comparable to what has been reported on BN substrates [19] with no signature of SOC enhancement. In contrast, for V BG > V TH , we found a giant enhancement of SOC (~17 meV). The combination of high charge mobility and large proximity induced SOC results in a gate-tunable spin Hall effect (SHE) even at RT, a crucial ingredient in realizing spintronics paradigms such as the spin FET [5] and potentially even the quantum spin Hall insulator [3] . Device structure and measurement configurations The fabrication of graphene/WS 2 heterostructure ( Fig. 1a ) devices starts with the standard dry transfer method [4] of single-layer graphene (SLG) onto atomically flat few layers of WS 2 (see Supplementary Fig. 1 ). Subsequently, e-beam lithography is used to form electrodes and pattern graphene into a Hall bar. Typical channel lengths and widths are L =3 μm and w =1 μm, respectively. A pair of electrodes is also created directly on WS 2 . An optical image of a typical final device is shown in Fig. 1b . Experiments were carried out in two different measurement configurations. In the conventional local four-terminal measurement configuration (Hall bar), current I 16 flows between contact 1 and contact 6 and a local voltage drop is measured between contact 2 and contact 4. In the non-local measurement configuration (H bar), the current I 23 flows between the pair of contact 2 and contact 3, and a non-local voltage V 45 is recorded across the neighbouring pair of contact 4 and contact 5 ( Fig. 1c ). All measurements were performed with standard a.c. lock-in technique at low frequencies in vacuum as a function of magnetic field ( B ), back-gate voltage ( V BG ) at both RT and liquid-Helium temperatures. In total, we have characterized 10 graphene/WS 2 devices. Here we discuss two representative devices and unless otherwise stated, the results shown are from device B. 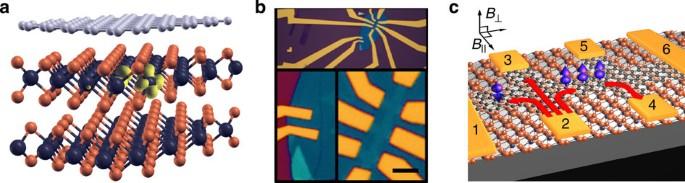Figure 1: Device characterization. (a) Schematics representation of a multilayer WS2/graphene heterostructure device. The highest unoccupied state of the sulphur vacancy is depicted in yellow, highlighting on the W atoms closest to the vacancy. W, S and C atoms are represented by dark grey, orange and light-grey spheres, respectively. (b) Optical micrograph of a completed device with multiple Hall bar junctions on G/WS2heterostructure and a two-terminal device on WS2. Scale bar, 2 μm. (c) Schematics for the local and non-local measurement configurations. Figure 1: Device characterization. ( a ) Schematics representation of a multilayer WS 2 /graphene heterostructure device. The highest unoccupied state of the sulphur vacancy is depicted in yellow, highlighting on the W atoms closest to the vacancy. W, S and C atoms are represented by dark grey, orange and light-grey spheres, respectively. ( b ) Optical micrograph of a completed device with multiple Hall bar junctions on G/WS 2 heterostructure and a two-terminal device on WS 2 . Scale bar, 2 μm. ( c ) Schematics for the local and non-local measurement configurations. 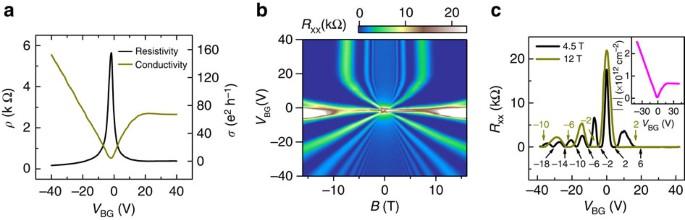Figure 2: Electronic transport measurement in graphene on WS2substrate. (a) Local resistivity (black lines) and conductivity (dark-yellow line) measurement as a function of back-gate voltage at 1.5 K. (b) Landau fan diagram of longitudinal resistance as a function of magnetic field and back-gate voltage. (c) Corresponding plots of longitudinal resistance as a function of back-gate voltage at constant magnetic fields. (Black and dark-yellow lines represent 4.5 T and 12 T, respectively.) Inset: carrier concentration as a function of applied back-gate voltage. Full size image Local charge transport Figure 2a shows the local conductivity σ of graphene on a WS 2 substrate as a function of V BG at T=1.5 K ( μ h ≈18,000 cm 2 V −1 s −1 ). While on the hole side σ is linear in V BG , on the electron side σ saturates above a threshold voltage V TH ≥15 V. A similar behaviour has been observed in all graphene on WS 2 devices and is absent, for example, in graphene on BN devices. We also performed two-terminal I – V measurements directly across WS 2 alone. To minimize any shunting of the current through the WS 2 , we use Cr/Au contacts (see Supplementary Figs 2 and 3 ). In such measurements, only an insulating response over the same V BG range is observed. Next, we discuss perpendicular magnetic-field ( B ⊥ )-dependent measurements as shown in Fig. 2b,c . From Hall effect measurements at low fields, we see that the origin of the conductance saturation on the electron side is due to the saturation of the charge density at ~7 × 10 11 cm −2 (inset, Fig. 2c ). The electron mobility above the saturation region is estimated to be μ e ≈24,750 cm 2 V −1 s −1 . The observation of such enhanced electronic mobility compared with graphene devices fabricated on SiO 2 substrate is due to improved substrate roughness and reduced fabrication residues left on graphene (see Supplementary Fig. 4 ). In high B ⊥ fields, this surprising saturation in conductivity result even alters the well-known Landau level (LL) fan diagram of graphene. This is clearly seen in the fan diagram where the longitudinal resistance, R XX , is recorded on a colour plot as a function of both V BG and the perpendicularly applied B ⊥ ( Fig. 2b ). For example, at B ⊥ =4.5 T, R XX versus V BG shows the regular integer quantum hall effect on the hole side with filling factor v =2, 6, 10, 14, 18, 22. However, on the electron side only the quantization for the first two LLs is observed. Since the LLs in graphene are not equally spaced in energy, it is possible to lock the graphene resistance even at the first LL for | B ⊥ |>10 T ( Fig. 2c ), making such graphene/WS 2 heterostructure potentially a suitable device for quantum resistance metrology [20] (see Supplementary Fig. 5 ). Figure 2: Electronic transport measurement in graphene on WS 2 substrate. ( a ) Local resistivity (black lines) and conductivity (dark-yellow line) measurement as a function of back-gate voltage at 1.5 K. ( b ) Landau fan diagram of longitudinal resistance as a function of magnetic field and back-gate voltage. ( c ) Corresponding plots of longitudinal resistance as a function of back-gate voltage at constant magnetic fields. (Black and dark-yellow lines represent 4.5 T and 12 T, respectively.) Inset: carrier concentration as a function of applied back-gate voltage. Full size image Non-local spin transport We now turn our attention to non-local transport measurements. This measurement technique is a powerful tool to detect spin-dependent transport phenomena that otherwise escape notice. Recently, this configuration has been, for example, used to detect Zeeman interaction-induced spin currents in graphene in the presence of an externally applied perpendicular magnetic field [21] , [22] . Balakrishnan et al. [8] , also implemented this geometry to demonstrate an enhancement of SOC in hydrogenated graphene by measuring spin precession in an in-plane magnetic field. We first discuss the RT non-local measurement of a graphene on SiO 2 device of comparable mobility ( μ ≈13.000 cm 2 V −1 s −1 ) ( Fig. 3a ). For such devices, the non-local resistance is symmetric around the Dirac peak and its magnitude over the entire back-gate bias range can be fully accounted for by an Ohmic leakage contribution [23] ,~ ρe − πL / w (dashed dotted fit to the data). In contrast, graphene on WS 2 substrates (devices B and C, Fig. 3b,c ) shows a non-local signal, which cannot be accounted for by an Ohmic contribution neither quantitatively nor qualitatively. First, the magnitude of the observed non-local signal is almost an order of magnitude larger than in graphene on SiO 2 samples. More importantly, we observe a strong electron–hole asymmetry in non-local resistance, which is completely absent in both graphene on SiO 2 and even in graphene on BN substrates (not shown). For instance, device B and device C have a non-local signal difference Δ R between the hole side and electron side of Δ R ~6.5 Ω and Δ R ~20 Ω, respectively. We find that there is a sample-to-sample variation of the non-local signal most likely due to a variation in the amount of the disorder in each sample (see Supplementary Fig. 6 ; Supplementary Table 1 ; Supplementary Note 1 ). However, the electron–hole asymmetry in the non-local signal is observed in all our graphene/WS 2 devices. Equally important, the onset of the asymmetry coincides with V TH at which the local conductivity saturates. Note that this asymmetry does rule out thermal effects as discussed in ref. 22 as the dominant effect. 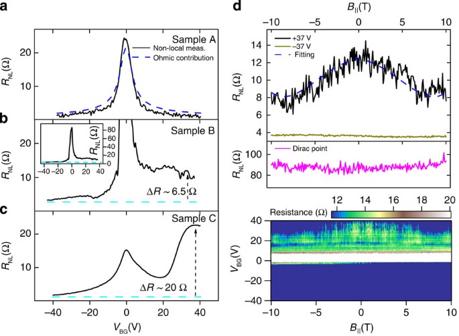Figure 3: Spin transport measurement in graphene on WS2substrate. (a) Non-local resistance measurement as a function of back-gate voltage at RT in a reference graphene/SiO2device. Sample A: (black line) with its calculated Ohmic contribution (blue line). (b,c) Non-local measurement for sample B and sample C at 1.5 K and RT, respectively. Inset (b) represents the complete data range of data from (b). (d) Fan diagram of non-local resistance as a function of in-plane magnetic field and back-gate voltage. Colour scale bar is adjusted to show between 12 and 20 Ω for clarification. Corresponding plots of non-local resistance as a function of in-plane magnetic field at constant back-gate voltages.(Black, pink and dark-yellow lines represent 37 V, 2 V (Dirac point (DP)) and −37 V, respectively). Figure 3: Spin transport measurement in graphene on WS 2 substrate. ( a ) Non-local resistance measurement as a function of back-gate voltage at RT in a reference graphene/SiO 2 device. Sample A: (black line) with its calculated Ohmic contribution (blue line). ( b , c ) Non-local measurement for sample B and sample C at 1.5 K and RT, respectively. Inset ( b ) represents the complete data range of data from ( b ). ( d ) Fan diagram of non-local resistance as a function of in-plane magnetic field and back-gate voltage. Colour scale bar is adjusted to show between 12 and 20 Ω for clarification. Corresponding plots of non-local resistance as a function of in-plane magnetic field at constant back-gate voltages. (Black, pink and dark-yellow lines represent 37 V, 2 V (Dirac point (DP)) and −37 V, respectively). Full size image In-plane magnetic-field dependence of non-local signal To determine the origin of the non-local signal, we applied a magnetic field B || in the plane of the device parallel to the current flow direction. Such Hanle spin precession measurements for device B as a function of V BG are summarized in Fig. 3d . Also, here we see a clear electron–hole asymmetry. The critical gate voltage at which the field dependence of the non-local signal changes markedly coincides again with V TH at which the conductance saturation is observed. For all V BG < V TH , the non-local signal is magnetic field independent. Two representative R NL versus B || traces at V BG =−37 V and V BG =2 V (Dirac point (DP)) are shown in Fig. 3d . On the other hand, for all V BG > V TH , the non-local signal shows a maximum at zero magnetic field and decreases with increasing | B || | with the onset of an oscillatory-type behaviour clearly visible for | B || |>8 T. Remarkably, the maximum observed change of the non-local signal Δ R ~6 Ω as a function of field is comparable to the difference observed in the non-local signal Δ R as a function of V BG ( Fig. 3b ). It is important to note that in this measurement configuration only a spin current can give rise to a magnetic-field-dependent signal [23] , [24] . Thus, the observation of the oscillatory magnetic-field-dependent signal directly proves the spin origin of the non-local signal. To assure there is no contribution from Joule heating and other spurious sources, we have also performed d.c. measurements with bias currents of few μA at both current polarities (see Supplementary Fig. 7 ). Both the magnitude and asymmetry of the non-local signal is identical in d.c. and a.c. measurements (see Supplementary Fig. 8 ). We are now ready to extract the spin transport parameters of our devices. For this, we fit the field dependence of the non-local signal using the following equation [23] : where γ is the spin Hall coefficient, w the width of the channel, ρ is the resistivity of the channel, ω B is the Larmor frequency, τ s is the spin relaxation time and λ s is the spin relaxation length. We obtain λ s =2 μm, τ s =5 ps. The strongly reduced τ s when compared with τ s of hydrogenated graphene devices [8] (~90 ps) and graphene spin valve devices [1] (~200 ps) is a direct consequence of the huge enhancement of SOC. However, having a high diffusion constant ( D ) in high-mobility graphene/WS 2 devices results in long λ s ), which is comparable to those observed in graphene-based spin valve devices [1] . We finally calculate the proximity SOC strength Δ SO . Since the dominant dephasing mechanism in SLG is Elliott–Yafet type [1] , [25] , we have (ref. 26 ) where ε F is the Fermi energy and τ P is the momentum relaxation time . Thus, we obtain a proximity SOC of 17.6 meV, which is even higher than that achieved by hydrogenating graphene [8] . With this, we identify the SHE and inverse SHE as the origin of the observed non-local signal. The latter is only possible because of the three orders of magnitude enhancement of the intrinsic SOC graphene when in proximity with WS 2 . SOC strength that is extracted from the temperature dependence of spin precession signal is at the same order with the value extracted above (see Supplementary Fig. 9 ). Low-field magnetoresistance measurements provided further evidence for a strong enhancement of the SOC for V BG > V TH . Here, we see at the same threshold voltage a transition from positive to negative magnetoresistance (see Supplementary Fig. 10 ). This transition from weak localization to weak anti-localization behaviour provides independent evidence for the proximity effect-induced SOC. Next, we discuss the origin of the proximity effect in more detail. Recently single sulphur vacancies have been observed in MoS 2 flakes using an atomic resolution direct imaging technique [27] , [28] . Similar structural defects are also expected for WS 2 crystals (see Supplementary Fig. 11 ). For this purpose, we characterized our chemical-vapour transport method-grown WS 2 crystals with X-ray photoelectron spectroscopy. 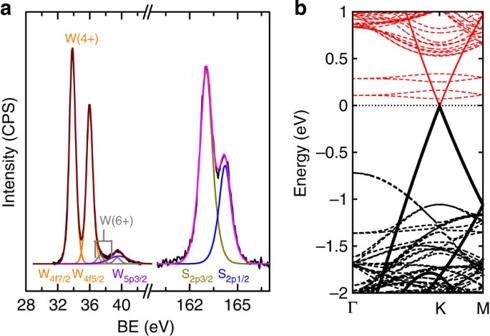Figure 4: X-ray photoelectron spectroscopy (XPS) measurement of WS2and DFT band tructure calculations. (a) High-resolution XPS of W4fand S2pcore levels. (b) Band structures of graphene and bulk WS2with a sulphur vacancy in bulk WS2(aligned with respect to the vacuum-level energy). In the latter, a rigid shift of 0.2 eV has been applied to the unoccupied states to correct the band gap to the experimental value32(compare withSupplementary Fig. 14). Figure 4a shows the X-ray photoelectron spectroscopy spectra of W 4f and S 2p from where we estimate a large concentration of sulphur vacancies of the order of 10 13 cm −2 (see Supplementary Fig. 12 ; Supplementary Note 2 ). This result shows that there are localized states in the gap of WS 2 , originating from sulphur vacancies. As a next step, we performed ab initio fully relativistic density functional theory (DFT) calculations to discuss the origin of these states and its relevance for the observed phenomena (see Supplementary Fig. 13 ; Supplementary Note 3 for the models of other possible sources of disorder). Our calculations for the band structure of the graphene/WS 2 interface show that the Dirac point of graphene is within the WS 2 band gap ( Fig. 4b ). The band structure of the interface is nearly a superposition of the band structures of the two moieties. The lowest conduction band of WS 2 is practically unchanged by the presence of graphene. Note that the proximity of WS 2 with or without vacancies does not induce any significant SOC in the graphene electronic bands (see Supplementary Fig. 14 ). Figure 4: X-ray photoelectron spectroscopy (XPS) measurement of WS 2 and DFT band tructure calculations. ( a ) High-resolution XPS of W 4f and S 2p core levels. ( b ) Band structures of graphene and bulk WS 2 with a sulphur vacancy in bulk WS 2 (aligned with respect to the vacuum-level energy). In the latter, a rigid shift of 0.2 eV has been applied to the unoccupied states to correct the band gap to the experimental value [32] (compare with Supplementary Fig. 14 ). Full size image A sulphur vacancy ( V S ) on the other hand, introduces a double unoccupied state in the top half of the band gap of bulk WS 2 . As shown in Fig. 4b , the Fermi level crosses only the graphene states, so the longitudinal electron transport uses graphene π states; the transverse electron transport involves tunnelling from graphene to the vacancy acceptor states and back to graphene. In fact, using , where ν F is the Fermi velocity (0.9 × 10 6 m s −1 ) calculated from the effective mass of charge carriers (see Supplementary Fig. 15 ) and n is the carrier concentration (7 × 10 11 cm −2 ) at V TH, we obtain ε F ~0.09 eV at V TH in good agreement with our theoretical estimate. The mid gap states originate on the vacancy dangling bonds and are localized on W. They have an unusually large spin splitting of about Δ E SO ~0.2 eV to which we assign the origin of the proximity SOC observed. The graphene electrons move from graphene to the vacancy states in WS 2 by quantum tunnelling. This tunnelling relies on the proximity of the wavefunction of the vacancy states to the graphene, which is characterized by hybridization energy V H . From the second-order perturbation theory (Δ E SO ≈ V H 2 /Δ SO ), the hybridization energy is estimated to be 0.059 eV. In conclusion, we have demonstrated the proximity-induced enhancement of otherwise weak SOC in graphene while simultaneously preserving its exceptionally high electronic quality. Our results in graphene/WS 2 heterostructures show SOC as high as 17 meV, which resulted in the observation of SHE even at RT. The SHE is further supported by performing the spin precession measurements. Our detailed theoretical and experimental analyses show that the origin of the proximity effect is intrinsic, due to the unavoidable defects in the WS 2 substrate. These defects not only strongly enhance the SOC but also act as a sink for electronic charges of graphene once the Fermi level aligns with these localized states, resulting in conductivity, which is independent of gate bias. Such enhancement of the SOC is crucial for the development of graphene-based spin FETs. WS 2 crystal growth Bulk crystals of 2H-WS 2 were grown by the chemical-vapour transport method using iodine as the transport agent. As-received WS 2 powder (Alfa Aesar, 99.9 purity %) was sealed in an ampoule of fused quartz. The ampoule was kept in a temperature gradient from 875 to 935 °C in a dual zone furnace for 1 week. WS 2 crystals grew on the cold end of the ampoule. Dry transfer method Transferring of graphene onto a WS 2 substrate process starts with the micromechanical exfoliation of SLG flake on a bilayer polymer stack. The bottom layer polymer is dissolved with its developer so that the remaining resist (poly(methyl methacrylate) (PMMA)) and the graphene flake are isolated from the supporting substrate. The resulting PMMA/graphene film is transferred onto previously exfoliated WS 2 crystal (the thickness of WS 2 substrates varied from 5 to 15 nm). During this process, the graphene surface to be transferred onto the WS 2 crystal surface never gets exposed to any solvent, resulting in ultra-clean interfaces. After the transfer process, the graphene surface that is contacted to the PMMA layer is annealed at 340 °C for 6 h in forming gas to remove the transfer residues. Hall bar structures are only fabricated in wrinkle, bubble-free regions. Electronic quality of graphene devices fabricated on different 2D crystals by employing this dry transfer method is discussed in ref. 29 . DFT calculations The fully relativistic DFT calculations were performed using the method described in ref. 30 . For the dispersion, we used the correction by Grimme [31] . Bulk WS 2 was modelled using a 4 × 4 × 1 supercell, with the experimental c/a ratio. The graphene/WS 2 monolayer interface was modelled in a supercell with 3 × 3 primitive cells of WS 2 and 4 × 4 primitive cells of graphene, with the respective lattice vectors aligned. How to cite this article : Avsar, A. et al. Spin–orbit proximity effect in graphene. Nat. Commun. 5:4875 doi: 10.1038/ncomms5875 (2014).